Spinel-type lithium cobalt oxide as a bifunctional electrocatalyst for the oxygen evolution and oxygen reduction reactions Development of efficient, affordable electrocatalysts for the oxygen evolution reaction and the oxygen reduction reaction is critical for rechargeable metal-air batteries. Here we present lithium cobalt oxide, synthesized at 400 °C (designated as LT-LiCoO 2 ) that adopts a lithiated spinel structure, as an inexpensive, efficient electrocatalyst for the oxygen evolution reaction. The catalytic activity of LT-LiCoO 2 is higher than that of both spinel cobalt oxide and layered lithium cobalt oxide synthesized at 800 °C (designated as HT-LiCoO 2 ) for the oxygen evolution reaction. Although LT-LiCoO 2 exhibits poor activity for the oxygen reduction reaction, the chemically delithiated LT-Li 1−x CoO 2 samples exhibit a combination of high oxygen reduction reaction and oxygen evolution reaction activities, making the spinel-type LT-Li 0,5 CoO 2 a potential bifunctional electrocatalyst for rechargeable metal-air batteries. The high activities of these delithiated compositions are attributed to the Co 4 O 4 cubane subunits and a pinning of the Co 3+/4+ :3d energy with the top of the O 2− :2p band. Oxygen electrochemistry plays a major role in energy conversion and storage devices, particularly in the field of fuel cells, metal-air batteries and water electrolysers [1] , [2] , [3] . The major challenge in metal-air batteries and water electrolysis is to design and develop economically feasible, earth-abundant, inexpensive, efficient electrocatalysts for the oxygen evolution reaction (OER) [4] . In nature, water electrolysis is performed by the photosystem II water-oxidizing complex containing CaMn 4 O x clusters that are capable of promoting water oxidation with significant turnover frequencies at low overpotentials [4] , [5] , [6] , [7] , [8] . However, it is difficult to use these naturally occurring enzymes in commercial electrochemical devices due to their instability under the operating conditions [9] . Precious-metal electrocatalysts such as Pt, IrO 2 and RuO 2 are normally employed, but their low abundance and high cost prohibit their practical use [10] . Pt exhibits inadequate OER activity due to the formation of the insulating platinum oxides. RuO 2 becomes unstable at high potentials due to the formation of higher-valent ruthenium oxides. IrO 2 is the best electrocatalyst so far for OER. Moreover, it is difficult to get both acceptable OER and oxygen reduction reaction (ORR) activities with the same material. Therefore, a burgeoning effort by chemists is to develop inexpensive materials with high electrocatalytic activity and stability for OER or preferably for both OER and ORR, but it remains a daunting scientific challenge. In addition, electrolysis of water is generally preferred in alkaline medium over acidic medium because of the less expensive materials for construction and less susceptibility to corrosion [11] , [12] , [13] . Transition metal oxides containing highly oxidized redox couples such as Ir 4+/6+ , Ru 4+/8+ , Co 3+/4+ , Ni 3+/4+ , Mn 3+/4+ and Fe 3+/4+ are known as active centres for OER. The electrochemical performance of oxides for OER follows the order, IrO 2 >RuO 2 >Co 3 O 4 and Ni-containing cobalt oxides>Fe, Pb, Mn containing oxides. Among the numerous low-cost oxides investigated, cobalt oxides are promising for both OER and ORR [14] , [15] , [16] , [17] , [18] and have been largely studied as stable electrocatalysts for OER in highly alkaline solutions [19] . For example, spinel NiCo 2 O 4 and Co 3 O 4 have been found by several groups to show good efficiency and long-term performance, but they underperform relative to IrO 2 (ref. 20 ). Co 3 O 4 nanoparticles have also been anchored onto suitable conducting supports to prevent the agglomeration of nanoparticles and thereby increase the electrocatalytic activity. Recently, Liang et al. [21] have used Co 3 O 4 nanocrystals anchored onto graphene, while Frei and co-workers [22] have developed efficient water oxidation electrocatalysts by supporting MnO x and Co 3 O 4 clusters on mesoporous silica scaffolds. Also, Kanan et al. [23] have used cobalt phosphate as an electrocatalyst for water oxidation. With an aim to develop highly active electrocatalysts based on earth-abundant elements for both OER and ORR, we focus here on LiCoO 2 as an electrocatalyst. LiCoO 2 has been intensively studied as a cathode material for lithium-ion batteries [24] . LiCoO 2 is known to exist in two forms as described below. The LiCoO 2 sample synthesized at high temperatures (~\n800 °C) has the α-NaFeO 2 structure (space group: ) in which the Li + and Co 3+ ions order on alternate {111} planes of the rock salt structure due to the large size and charge differences between the Li + and Co 3+ ions [25] . We designate this high-temperature form as HT-LiCoO 2 . In contrast, the LiCoO 2 sample synthesized at lower temperatures (~\n 400 °C) adopts a lithiated spinel structure {Li 2 } 16c [Co 2 ] 16d O 4 in which the Co 3+ ions occupy all the 16d octahedral sites, while the Li + ions occupy all the 16c octahedral sites of the spinel framework (space group: Fd3m ) [26] . We designate this low-temperature form as LT-LiCoO 2 . In this paper, we compare the activities of LT-LiCoO 2 and HT-LiCoO 2 having the same composition but different structures for OER in alkaline medium. LT-LiCoO 2 and HT-LiCoO 2 , both consisting of Co 3+ ions, offer a unique platform to explore the structure-activity relationship for OER. While LT-LiCoO 2 consists of the cubane-like cubic Co 4 O 4 units, HT-LiCoO 2 consists of LiCo 3 O 4 units. Also, the changes in the surface structure of LT-LiCoO 2 and its OER activity as a function of the firing time and temperature around 400 °C are presented. We also compare the OER and ORR activities of chemically delithiated LT-Li 1−x CoO 2 as a function of lithium content (0≤x≤0.5) and the oxidation state of Co with an aim to utilize it as a bifunctional electrocatalyst for OER and ORR. Bulk and surface structures Both the atomic and electronic structures, particularly on the surface under the electrochemical operating conditions, play a critical role in imparting the electrocatalytic activity for OER and ORR. 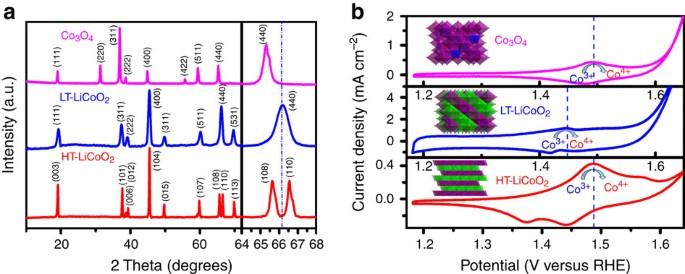Figure 1: X-ray diffraction patterns and electrochemical behaviour of electrocatalysts. (a) X-ray diffraction patterns of Co3O4, LT-LiCoO2and HT-LiCoO2, illustrating the splitting of the (440) reflection in the cubic spinel LT-LiCoO2into (108) and (110) reflections in the rhombohedral-layered LT-LiCoO2as shown in the expanded region of 2θ=64–68°. (b) Cyclic voltammograms of Co3O4,LT-LiCoO2and HT-LiCoO2in 0.1 M KOH at scan rate of 5 mV s−1. The purple, blue and green colours in the structures shown in the insets ofbrefer, respectively, to the polyhedra of Co3+, Co2+and Li+ions. Figure 1a shows the X-ray diffraction patterns of LT-LiCoO 2 , HT-LiCoO 2 and Co 3 O 4 . While the LT-LiCoO 2 synthesized at 400 °C shows a single reflection around 2θ≈63° corresponding to the {440} plane of the cubic lithiated spinel ( Fd3m ), it splits into the (108) and (110) reflections of the layered HT-LiCoO 2 structure ( ) on heating to 800 °C [27] , [28] , [29] , [30] . Also, the (220) reflection present in Co 3 O 4 is absent in LT-LiCoO 2 due to the absence of ions with high scattering power in the 8a tetrahedral sites of the spinel lattice in LT-LiCoO 2 . Co 3 O 4 has the cubic spinel structure with a cation distribution of (Co 2+ ) 8a [Co 2 3+ ] 16d O 4 in which all the Co 3+ ions occupy the 16d octahedral sites, while all Co 2+ ions occupy the 8a tetrahedral sites. Supplementary Fig. 1 shows the Rietveld refinement of the X-ray diffraction data of LT-LiCoO 2 and HT-LiCoO 2 along with Co 3 O 4 . The observed and calculated patterns match well with each other, validating the cubic lithiated spinel structure of LT-LiCoO 2 . The structural parameters obtained from the Rietveld refinement are given in Supplementary Table 1 . Figure 1: X-ray diffraction patterns and electrochemical behaviour of electrocatalysts. ( a ) X-ray diffraction patterns of Co 3 O 4 , LT-LiCoO 2 and HT-LiCoO 2 , illustrating the splitting of the (440) reflection in the cubic spinel LT-LiCoO 2 into (108) and (110) reflections in the rhombohedral-layered LT-LiCoO 2 as shown in the expanded region of 2θ=64–68°. ( b ) Cyclic voltammograms of Co 3 O 4, LT-LiCoO 2 and HT-LiCoO 2 in 0.1 M KOH at scan rate of 5 mV s −1 . The purple, blue and green colours in the structures shown in the insets of b refer, respectively, to the polyhedra of Co 3+ , Co 2+ and Li + ions. 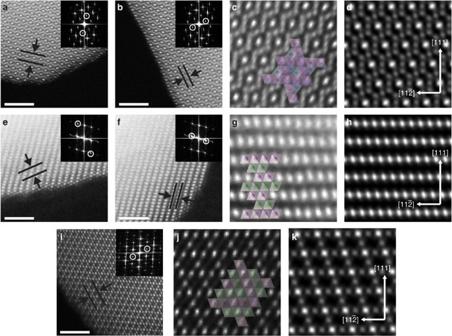Figure 2: Aberration-corrected HAADF-STEM images of electrocatalyts. HAADF-STEM images of (a–d) Co3O4, (e–h) HT-LiCoO2and (i–k) LT-LiCoO2viewed down thezone axis, showing the surface structure at the (a,e,i) {001} plane and (b,f) {111} plane. These surface planes are indicated by black bars and arrows in the image and circles in the inset fast Fourier transform’s (FFT’s). The unit cells for each composition with octahedral and tetrahedral arrangements are overlaid on higher magnification images that have been deconvoluted to reduce noise in (c,g,j)44. The blue, purple and green atoms refer, respectively, to Co2+, Co3+and Li+. The simulated STEM images are shown in (d,h,k). To facilitate a comparison of the three materials, the deconvoluted and simulated images have been rotated relative to the STEM images, so that all the {111} planes lie on the horizontal axis. Scale bar, 2 nm. Full size image Figure 2 shows the aberration-corrected high angular annular dark-field scanning transmission electron microscopy (STEM) images of the three samples, viewed down the zone axis. The atomic arrangement in the Co 3 O 4 particle matches that expected for the spinel lattice with the space group , where the Co 3+ ions occupy the octahedral sites and Co 2+ ions occupy the tetrahedral sites ( Fig. 2c,d ). The particle maintains this structure all the way to the surface on both the {001} and {111} planes ( Fig. 2a,b , respectively). As a comparison, the surfaces of the {001} and the {111} planes in HT-LiCoO 2 are shown in Fig. 2e,f . The overall structure matches that of a trigonal lattice with the space group ( Fig. 2g,h ). For ease of comparison, we will use the cubic system, which is the most basic structure of HT-LiCoO 2 , for the notation of the planes in both the figures and the discussion of HT-LiCoO 2 . The bulk structure of HT-LiCoO 2 is maintained all the way to the surface on the {111} planes ( Fig. 2f ), but shows some variation for a few layer of the {001} surface ( Fig. 2e ). At this surface, there are some bright atomic columns of Co that appear in the Li layers, suggesting that some Co might have moved into the lithium layer at the {001} cubic surface. The bulk structure of LT-LiCoO 2 is shown in Fig. 2i , and it indicates that the structure corresponds to a spinel lattice with the space group and Co and Li occupying, respectively, all the 16d and 16c octahedral sites ( Fig. 2j,k ). The structure of the {001} planes is maintained all the way to the surface ( Fig. 2i ). The structure of the {111} planes at the surface, however, is modified under certain synthesis conditions ( Fig. 3 ). For example, for a firing temperature of 370 °C for 7 days, the spinel structure is maintained all the way to the {111} surface ( Fig. 3a ). For firing temperatures of 385 and 400 °C for 7 days, however, a few atomic layers of the {111} surface planes have transformed to the layered HT-LiCoO 2 ( Fig. 3b,c ). In contrast, for a firing temperature of 400 °C for 4 days, only the first layer has transformed to the layered HT-LiCoO 2 phase ( Fig. 3d ). Figure 2: Aberration-corrected HAADF-STEM images of electrocatalyts. HAADF-STEM images of ( a – d ) Co 3 O 4 , ( e – h ) HT-LiCoO 2 and ( i – k ) LT-LiCoO 2 viewed down the zone axis, showing the surface structure at the ( a , e , i ) {001} plane and ( b , f ) {111} plane. These surface planes are indicated by black bars and arrows in the image and circles in the inset fast Fourier transform’s (FFT’s). The unit cells for each composition with octahedral and tetrahedral arrangements are overlaid on higher magnification images that have been deconvoluted to reduce noise in ( c , g , j ) [44] . The blue, purple and green atoms refer, respectively, to Co 2+ , Co 3+ and Li + . The simulated STEM images are shown in ( d , h , k ). To facilitate a comparison of the three materials, the deconvoluted and simulated images have been rotated relative to the STEM images, so that all the {111} planes lie on the horizontal axis. Scale bar, 2 nm. 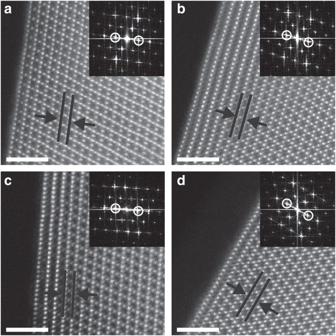Figure 3: Aberration-corrected HAADF-STEM images of LT-LiCoO2. HAADF-STEM images of LT-LiCoO2viewed down thezone axis showing the atomic structure of the {111} planes at the surface for samples prepared at (a) 370 °C for 7 days, (b) 385 °C for 7 days, (c) 400 °C for 7 days and (d) 400 °C for 4 days. These surface planes are indicated by black bars and arrows in the image and circles in the inset fast Fourier transform ‘s (FFT’s). The scale bars are 2 nm. Full size image Figure 3: Aberration-corrected HAADF-STEM images of LT-LiCoO 2 . HAADF-STEM images of LT-LiCoO 2 viewed down the zone axis showing the atomic structure of the {111} planes at the surface for samples prepared at ( a ) 370 °C for 7 days, ( b ) 385 °C for 7 days, ( c ) 400 °C for 7 days and ( d ) 400 °C for 4 days. These surface planes are indicated by black bars and arrows in the image and circles in the inset fast Fourier transform ‘s (FFT’s). The scale bars are 2 nm. Full size image Electrochemical behaviour Cyclic voltammograms (CVs) recorded for all the three electrocatalysts under the same experimental conditions at a scan rate of 5 mV s −1 are presented in Fig. 1b . The enlarged CVs and the CVs recorded for an extended number of cycles are shown in Supplementary Fig. 2 . The CV of Co 3 O 4 is characterized by a single anodic peak before the OER and a single cathodic peak, which have been attributed to the quasi-reversible redox couple (CoO 2 /CoOOH) occurring on Co 3 O 4 surface [15] , [31] . The CV of HT-LiCoO 2 differs considerably from that of Co 3 O 4. HT-LiCoO 2 shows two peaks during the anodic process and two peaks during the cathodic process, and the redox peaks become more pronounced during extended CV cycling ( Supplementary Fig. 2b ). Unlike in Co 3 O 4 , the Co 3+/4+ oxidation/reduction in HT-LiCoO 2 is accompanied by lithium extraction/insertion. Also, HT-LiCoO 2 is known to insert protons into the lattice during chemical delithiation (with NO 2 BF 4 even in acetonitrile medium) for x>0.5 in HT-Li 1−x CoO 2 and transform from the O3-layered structure to the P3-layered structure [32] , [33] . While the Li + ions are in octahedral sites in the O3 structure, the Li + /H + ions are in prismatic sites in the P3 structure. Thus, the occurrence of two peaks during the anodic or cathodic process is due to the extraction/insertion of Li + /H + into two different crystallographic sites. It should be noted that the second anodic peak is weak and it becomes invisible at higher scan rates (for example, 20 mV s −1 ), possibly due to the slow kinetics associated with the extraction/insertion of Li + /H + from/into the prismatic sites. LT-LiCoO 2 also shows two anodic peaks ( Fig. 1b and Supplementary Fig. 2 ), but the second peak is much weaker even at a slow scan rate of 5 mV s −1 . This is because the lithium diffusion rate is much slower in LT-LiCoO 2 , which has a lithiated spinel structure formed at low temperatures, possibly with defects, compared with that in HT-LiCoO 2 that has a well-formed, well-ordered layered structure [30] , [34] . In addition, LT-LiCoO 2 may also undergo structural transformations at deep lithium extraction, involving possibly proton insertion, due to the instability at high Co 4+ contents. Thus, the occurrence of two peaks is due the extraction/insertion of Li + /H + from/into two different lattice sites. It is clear that the anodic peak corresponding to lithium extraction is sensitive to diffusion coefficient and the CV scan rate [35] . Furthermore, the anodic peak in LT-LiCoO 2 occurs at a lower potential (1.43 V) than that in HT-LiCoO 2 (1.49 V), despite the same composition and oxidation state of Co, reflecting the influence of crystal structure (spinel-like versus layered). Supplementary Table 2 gives the potential and redox couples for various electrocatalysts. Nocera’s group [36] has pointed out that the structurally strained, unstable Co 4+ species on the surface acts as an intermediate species for OER. They have also demonstrated Co 4+ active site formation by EPR during the OER conditions. Rasiyah et al. [37] have shown a relationship between the onset potential for OER and the potential of the lower oxide/higher oxide couple. For example, the redox couples of IrO 2 and RuO 2 occurring at lower potentials results in lower OER onset potentials for both compositions [37] . Thus, the occurrence of the Co 3+ /Co 4+ redox couple peak at a lower potential in LT-LiCoO 2 leads to lower OER onset potential compared with those of HT-LiCoO 2 and Co 3 O 4 ( Supplementary Table 2 ). The electrocatalytic activities of Co 3 O 4 , LT-LiCoO 2 , HT-LiCoO 2 and the conventional IrO 2 samples for OER were studied by linear sweep voltammetry in oxygen-saturated 0.1 M KOH solution at a scan rate of 20 mV s −1 . The mass normalized OER activities ( Fig. 4a ) of the samples increase in the order: HT-LiCoO 2 <Co 3 O 4 <IrO 2 <LT-LiCoO 2 . Among the electrocatalysts studied, the layered HT-LiCoO 2 sample exhibits the lowest OER activity, close to that of the well-studied Co 3 O 4 , while the LT-LiCoO 2 sample (prepared at 400 °C for 7 days) exhibits the highest OER activity that is even slightly better than that of the well-known IrO 2 electrocatalyst. However, IrO 2 shows a lower OER onset potential compared with LT-LiCoO 2 . Also, LT-LiCoO 2 exhibits much higher OER activity than the best-studied perovskite oxide Ba 0.5 Sr 0.5 Co 0.8 Fe 0.2 O 3−δ (refs 2 , 38 ) ( Supplementary Table 3 ). Linear sweep voltammograms cycles of LT-LiCoO 2 in 0.1 M KOH at pH=13 are shown in Supplementary Fig. 3 . Interestingly, the OER activity is found to increase gradually, approach a stable value after 100 cycles, and then decrease slowly after 200 cycles. Anodic linear scanning voltammograms for OER on the LT-LiCoO 2 electrodes at different sweep rates are shown in Supplementary Fig. 4 .The current density increases with increasing sweeping rate. The high OER activity of LT-LiCoO 2 is consistent with the high activity observed recently for the photocatalytic oxidation of water [39] . To understand the OER activities further, the Tafel plot analysis is shown in Supplementary Fig. 5 . The Tafel slope observed for Co 3 O 4 (67 mV dec −1 ) is in good agreement with those reported for Co 3 O 4 nanocrystals on a graphene support [31] . The LT-LiCoO 2 and LT-Li 0.5 CoO 2 samples exhibit smaller Tafel slopes of, respectively, 52 and 60 mV dec −1 than Co 3 O 4 and HT-LiCoO 2 , which is consistent with the reported values of 63 mV dec −1 for lithium-doped Co 3 O 4 in alkaline electrolytes [37] . Also, LT-LiCoO 2 and LT-Li 0.5 CoO 2 exhibit higher exchange current densities than Co 3 O 4 and HT-LiCoO 2 . The higher exchange current density and smaller Tafel slope of LT-LiCoO 2 attest to its good electrocatalytic activity for OER. 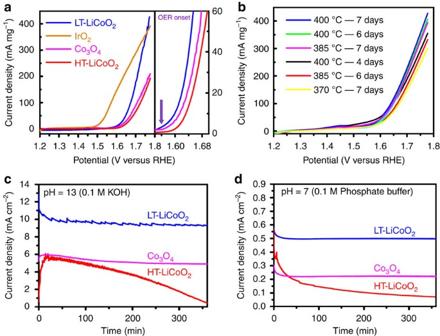Figure 4: OER Performances of the electrocatalysts. (a) Linear sweep voltammograms of LT-LiCoO2, IrO2, Co3O4and HT-LiCoO2at a scan rate of 20 mV s−1at 1,600 r.p.m. in 0.1 M KOH at pH=13, with an expanded region shown on the right. (b) Effect of firing temperature and time on the OER activity of LT-LiCoO2. (c) Chronoamperometry of LT-LiCoO2, Co3O4and HT-LiCoO2recorded at 1.7 V and 1,600 r.p.m. in 0.1 M KOH (pH=13). (d) Chronoamperometry of LT-LiCoO2, Co3O4and HT-LiCoO2recorded at 1.7 V and 1,600 r.p.m. in 0.1 M phosphate buffer solution (pH=7). Some fluctuations observed in the data points at high pH compared with the neutral pH arise from the formation of bubbles on the surface of the electrode. The glassy carbon RDE electrodes were held under rotation at 1,600 r.p.m. during the course of the experiment in order to effectively remove the bubbles formed during the OER. All activities are IR-corrected and normalized to the mass activity. Figure 4: OER Performances of the electrocatalysts. ( a ) Linear sweep voltammograms of LT-LiCoO 2 , IrO 2 , Co 3 O 4 and HT-LiCoO 2 at a scan rate of 20 mV s −1 at 1,600 r.p.m. in 0.1 M KOH at pH=13, with an expanded region shown on the right. ( b ) Effect of firing temperature and time on the OER activity of LT-LiCoO 2 . ( c ) Chronoamperometry of LT-LiCoO 2 , Co 3 O 4 and HT-LiCoO 2 recorded at 1.7 V and 1,600 r.p.m. in 0.1 M KOH (pH=13). ( d ) Chronoamperometry of LT-LiCoO 2 , Co 3 O 4 and HT-LiCoO 2 recorded at 1.7 V and 1,600 r.p.m. in 0.1 M phosphate buffer solution (pH=7). Some fluctuations observed in the data points at high pH compared with the neutral pH arise from the formation of bubbles on the surface of the electrode. The glassy carbon RDE electrodes were held under rotation at 1,600 r.p.m. during the course of the experiment in order to effectively remove the bubbles formed during the OER. All activities are IR-corrected and normalized to the mass activity. Full size image The large difference between the OER performances of LT-LiCoO 2 and HT-LiCoO 2 again reflects the importance of structural features for OER, for example, Co 4 O 4 cubane units in LT-LiCoO 2 versus LiCo 3 O 4 units in HT-LiCoO 2 . Finally, despite the same spinel framework, the spinel Co 3 O 4 sample shows much lower activity (similar to that of layered LT-LiCoO 2 ) than the lithiated spinel LT-LiCoO 2 sample. This difference may be due to the presence of Co 2+ ions in the 8a tetrahedral sites of Co 3 O 4 and the difficulty of oxidizing the tetrahedral-site Co 2+ ions before oxidizing the octahedral-site Co 3+ ions to Co 4+ . This again reflects the importance of surface atomic arrangements and electronic structures for OER. Figure 4b compares the OER activities of the LT-LiCoO 2 samples prepared under various conditions. As seen, the sample fired at 400 °C for 7 days shows the highest OER activity, while the sample fired at 370 °C for 7 days shows the lowest OER activity, but all of them exhibit higher activity than HT-LiCoO 2 . The lowest activity of the sample fired at 370 °C for 7 days could be due to the incomplete solid state-reaction and the unreacted raw materials on the surface. For a given firing temperature of 400 °C, the OER activity increases with increasing firing time from 4–5 to 7 days. Similarly, for a given firing time of 7 days, the OER activity increases with increasing firing temperature from 370–385 to 400 °C. These observations reflect the importance of completing the solid-state reaction and realizing the optimum surface structures favourable for OER. It is possible that the presence of a few layers of layered HT-LiCoO 2 on the surface of LT-LiCoO 2 and the consequent surface strains arising from slight lattice mismatch between the two structures may play a role in maximizing the OER activity; future in-depth investigation could shed more light on this. The long-term stability of the electrocatalysts is a critical factor for them to be employed in practical devices. Accordingly, the durability of the electrocatalysts for OER at an applied potential of 1.7 V at pH=13 and 7 was evaluated by chronoamperometry ( Fig. 4c,d ). The Co 3 O 4 sample is stable both in alkaline (pH=13) and neutral (pH=7) media as seen in Fig. 4c,d . Interestingly, while the layered HT-LiCoO 2 shows a decrease in OER activity with time in alkaline medium ( Fig. 4c ) and even in neutral medium ( Fig. 4d ), the lithiated spinel LT-LiCoO 2 is stable in both neutral and alkaline (pH=13) media with time (6 h) as seen in Fig. 4c,d . Clearly, in addition to the higher OER activity, the spinel LT-LiCoO 2 offers stability advantages compared with the layered HT-LiCoO 2 , in spite of a slightly larger surface area for LT-LiCoO 2 (9.6 m 2 g −1 ) compared with that for HT-LiCoO 2 (1.7 m 2 g −1 ); the surface area of LT-LiCoO 2 was similar to that of Co 3 O 4 (9.4 m 2 g −1 ). The stability differences again reflect the importance of atomic arrangements for stable OER activity. Chemically delithiated LT-Li 1−x CoO 2 For an electrocatalyst to be employed in rechargeable metal-air batteries, it should display both acceptable OER and ORR activities. Accordingly, the ORR activity of LT-LiCoO 2 was evaluated with a rotating-disk electrode (RDE) in O 2 -saturated 0.1 M KOH electrolyte. As seen in Fig. 5a , LT-LiCoO 2 shows poor ORR activity, which is worse than that of Co 3 O 4 . Considering that samples with mixed-valent Co 3+/4+ are known to generally exhibit high ORR activities [40] , lithium was extracted chemically from LT-LiCoO 2 with the oxidizer NO 2 BF 4 in acetonitrile medium [33] , [41] to give LT-Li 1−x CoO 2 (0≤x≤0.5) with mixed-valent Co 3+/4+ . Interestingly, the ORR activity of the delithiated LT-Li 1−x CoO 2 samples increases with decreasing lithium content and the LT-Li 0.5 CoO 2 sample exhibits the highest ORR activity in Fig. 5a . 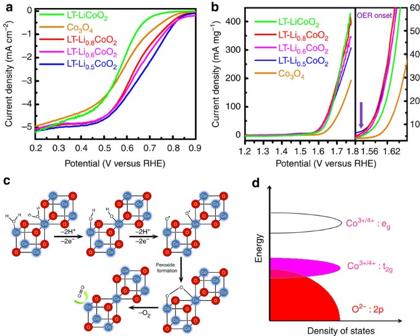Figure 5: Electrochemical performances of delithiated LT-Li1−xCoO2electrocatalysts. (a) ORR activities of LT-Li1−xCoO2for 0≤x≤0.5 in comparison with Co3O4in 0.1 M KOH at 1,600 r.p.m. (b) OER activities of LT-Li1−xCoO2for 0≤x≤0.5 in 0.1 M KOH at 1,600 r.p.m. with an expanded region shown on the right. (c) Mechanism of OER on Co4O4cubane units in LT-LiCoO2. (d) Qualitative one-electron energy diagram of Li1−xCoO2, illustrating the pinning of the Co3+/4+:3d energy with the top of the O2−:2p band. Figure 5b displays the OER activities of the delithiated LT-Li 1−x CoO 2 samples, and the OER activity decreases slightly with decreasing lithium content. Nevertheless, the LT-Li 0.5 CoO 2 sample exhibits 1.5 times higher OER activity than the Co 3 O 4 sample. However, the delithiated LT-Li 0.5 CoO 2 sample exhibits slightly lower stability than LT-LiCoO 2 at pH=13 ( Supplementary Fig. 6a ). The ambient-temperature chemical delithiation offers an approach to vary the d -electron count on the transition-metal ion and explore its influence on ORR and OER activities. In addition, the LT-LiCoO 2 sample shows good long-term stability for 20 h ( Supplementary Fig. 6a ), better than the highest reported for perovskite Ba 0.5 Sr 0.5 Co 0.8 Fe 0.2 O 3−δ (refs 2 , 38 ). Thus, the chemically delithiated spinel-type LT-Li 0.5 CoO 2 exhibits a combination of high ORR and OER activities with good stability, demonstrating it to be an excellent bifunctional electrocatalyst. Figure 5: Electrochemical performances of delithiated LT-Li 1−x CoO 2 electrocatalysts. ( a ) ORR activities of LT-Li 1−x CoO 2 for 0≤x≤0.5 in comparison with Co 3 O 4 in 0.1 M KOH at 1,600 r.p.m. ( b ) OER activities of LT-Li 1−x CoO 2 for 0≤x≤0.5 in 0.1 M KOH at 1,600 r.p.m. with an expanded region shown on the right. ( c ) Mechanism of OER on Co 4 O 4 cubane units in LT-LiCoO 2 . ( d ) Qualitative one-electron energy diagram of Li 1−x CoO 2 , illustrating the pinning of the Co 3+/4+ :3d energy with the top of the O 2− :2p band. Full size image We have successfully demonstrated that the non-noble metal LT-LiCoO 2 synthesized at 400 °C exhibits superior OER activity, even slightly better than that of IrO 2 . This is the highest mass activity reported to date for a non-noble-metal electrocatalyst or a noble-metal catalyst. For a material to have good OER activity, it should have high electronic conductivity and great affinity for adsorbed OH − intermediates. For example, IrO 2 is known to be the most active and stable electrocatalyst for OER in acid and alkaline media due to its interesting electronic structure and metallic conductivity. The OER reaction with IrO 2 involves an oxidation of low-spin Ir 4+ :5d 5 (t 2g 5 e g 0 ) ions to Ir 6+ :5d 5 (t 2g 3 e g 0 ) on the surface. The decrease in crystal field stabilization energy (CFSE) during this process has been suggested to make Ir 6+ unstable [37] , favouring a facile OER reaction. Similarly, the high OER activity of LT-LiCoO 2 could be related to (i) the decrease in CFSE during the oxidation of low-spin Co 3+ :3d 6 (t 2g 6 e g 0 ) ions to Co 4+ :3d 5 (t 2g 5 e g 0 ) on the surface or the formation of intermediate-spin Co 3+ (t 2g 5 e g 1 ) ions on the surface under the OER conditions in contact with the electrolyte and (ii) the high (possibly metallic) conductivity arising from the partially filled t 2g orbitals of Co 4+ or intermediate-spin Co 3+ ions across the shared octahedral edges of the spinel framework. In addition, the high OER activity of LT-LiCoO 2 may be related to the Co 4 O 4 cubane-like structure similar to that found in natures’ water oxidation catalyst CaMn 4 O x [4] , [5] , [6] , [7] , [8] as illustrated in Fig. 5c and the pinning of the Co 3+/4+ :3d energy with the top of the O 2− :2p band as shown in Fig. 5d . Direct coupling on adjacent Co 3+/4+ ions across a large number of cubic faces can facilitate the formation of O–O bonds easily as illustrated in Fig. 5c , leading to an easier release of oxygen [42] , [43] . Similar mechanisms could occur with other spinel OER electrocatalysts as well, but the pinning of the Co 3+/4+ :3d energy with the top of the O 2− :2p band may play a key role. In contrast, the presence of LiCo 3 O 4 units rather than Co 4 O 4 units in HT-LiCoO 2 diminishes such coupling across the cubic faces, resulting in lower OER activity. Furthermore, the surface atomic arrangement of LT-LiCoO 2 is sensitive to the firing temperature (around 400 °C) and time. The transformation of surface layers from a spinel-type arrangement to a layer-type arrangement with increasing firing temperature or time reveals that the spinel LT-LiCoO 2 is metastable (kinetically stabilized due to the lack of adequate ionic diffusion), and it tends to transform to the thermodynamically more stable HT-LiCoO 2 , by starting on the surface, with increasing firing temperature and time. Although LT-LiCoO 2 with single-valent Co 3+ ions exhibits poor ORR activity, the ORR activity could be drastically increased by chemically extracting lithium from LT-LiCoO 2 to give LT-Li 1−x CoO 2 . The extraction of lithium from LT-LiCoO 2 results in an oxidation of part of the Co 3+ ions to Co 4+ ions and a creation of mixed-valent Co 3+/4+ ions. The strong covalency arising from a pinning of the Co 3+/4+ :3d states with the top of the O 2− :2p band as shown in Fig. 5d along with the high electronic conductivity arising from the partially filled Co 3+/4+ :t 2g band across the shared edges of the 3-dimensional spinel framework lead to high ORR activity on extracting lithium from LT-LiCoO 2 . Thus, the partially delithiated LT-Li 0.5 CoO 2 , which could actually be a normal, ideal spinel (Li) 8a [Co 2 ] 16d O 4 , with mixed-valent Co 3+/4+ , offers a combination of high ORR and OER activities. Overall, the spinel-type delithiated LT-Li 0.5 CoO 2 behaves as a bifunctional electrocatalyst for OER and ORR in electrochemical devices such as rechargeable lithium-air batteries. Moreover, the chemical delithiation approach presented here to vary the number of d electrons on the transition-metal ion without changing the structure could be explored systematically with other compositions in the future (i) to correlate the d-electron count to ORR and OER activities and (ii) to develop a better understanding of the catalytic mechanisms of ORR and OER. Synthesis and characterization IrO 2 was purchased from Alfa Aesar. The lithiated spinel LT-LiCoO 2 samples were synthesized by a solid-state reaction of stoichiometric amounts of Li 2 CO 3 and Co 3 O 4 at 370–400 °C for various durations (4–7 days), followed by slow furnace cooling. The layered HT-LiCoO 2 sample was synthesized by solid-state reaction of stoichiometric amounts of Li 2 CO 3 and Co 3 O 4 at 800 °C for 24 h, followed by slow furnace cooling. The samples were characterized by X-ray diffraction with Cu Kα radiation. A Rietveld refinement of the X-ray diffraction data was carried out with the FullProf program. Multi-point Brunauer–Emmett–Teller (BET) surface areas of the samples were collected with an automatic nitrogen gas sorption analyser (NOVA 2000, Quantachrome) using physical adsorption at 77 K. Chemical extraction of lithium from LT-LiCoO 2 was carried out with a Schlenk line under argon atmosphere at room temperature with the oxidizer NO 2 BF 4 in acetonitrile medium [41] : LT-LiCoO 2 +xNO 2 BF 4 →LT-Li 1−x CoO 2 +xLiBF 4 +xNO 2 (1) The amount of lithium extracted was controlled by altering the amount of NO 2 BF 4 in the reaction medium. Typically, 200 mg of LT-LiCoO 2 was reacted with a specific amount of NO 2 BF 4 in 20 ml of anhydrous acetonitrile. After reacting for 1 day, the product formed was washed several times with acetonitrile to remove the byproduct LiBF 4 and then dried in an air oven at 100 °C. The lithium content in the delithiated sample was analysed by inductively coupled plasma (ICP) analysis. For STEM analysis, the powders were suspended in isopropanol, sonicated and placed onto a lacey carbon grid. The samples thus prepared were imaged on a JEOL ARM200F TEM/STEM equipped with a CEOS corrector (CEOS GmbH, Heidelberg, Ger.) for the illuminating lenses and a high-angle annular dark-field detector. Some of the high-resolution STEM images were deconvoluted using the maximum entropy method implemented by Ishizuka and Abe [44] . To simulate the STEM images, atomic models were created in Diamond 3.2i and exported to the high-resolution electron microscopy simulation suite, which is a TEM/STEM simulation software package based on the fast Fourier transform multislice technique [45] . For all the compositions, the multislice simulations were carried out assuming a step scanning size of 0.2 Å (less than the distance to be resolved) and a minimum slice thickness of 1.0 Å. The Debye-Waller factor (B), which is related to the mean square of the thermal displacement of an atom from its equilibrium position, was taken from the literature. In particular, the structures and B values for each atomic position were taken from the following: the crystal structure and temperature factors were taken from Meza et al. [46] for Co 3 O 4 , from our X-ray diffraction data with temperature factors all set to one for LT-LiCoO 2 , and from Rosolen et al. [47] for HT-LiCoO 2 . Electrochemical measurements Typically, 16 mg of the electrocatalyst sample and 3.2 mg of carbon black were dispersed in 8 ml of ethanol/water (1:1 ratio) and 73.2 μl of 5% Nafion solution by ultrasonication for 30 min to form a homogeneous catalyst ink. The catalyst ink was then coated onto the RDE (0.196 cm 2 ) at a loading of 0.25 mg oxide cm −2 disk and dried at room temperature. Before the coating of the catalyst, the glassy carbon electrode (5 mm diameter) was polished with Al 2 O 3 paste (0.05 μm) and washed ultrasonically with double-distilled water. All the electrochemical measurements were performed with a saturated calomel electrode as the reference electrode and a platinum foil counter electrode at a scan rate of 20 mV s −1 in 0.1 M KOH by purging a slow stream of purified oxygen gas towards the working electrode. The rotation speed of RDE was 1,600 r.p.m. for all measurements. Infrared (current × internal resistance) compensation was applied to linear sweep voltammetry experiments using the Nova software supplied with the Autolab cyclic voltammetry instrument. All potentials reported in this paper are relative to the reversible hydrogen electrode. The mass activity was normalized to the loading of the oxide catalyst. How to cite this article: Maiyalagan, T. et al. Spinel-type lithium cobalt oxide as a bifunctional electrocatalyst for the oxygen evolution and oxygen reduction reactions. Nat. Commun. 5:3949 doi: 10.1038/ncomms4949 (2014).